High strain rate deformation of layered nanocomposites Blast and ballistic impacts induce strong material nonlinearity and multiple complex, interacting deformation and failure mechanisms. Jet engine turbine blades are frequently damaged by high-speed collisions with solid particles entrained with the air, such as ice particles, hailstones and sand dust [1] , [2] , and satellites and spacecraft also suffer hypersonic damage by impact of minute particles such as micrometeorites and space debris [3] . All of these situations rely on material performance as critical to safety and survival. Although such high strain rate phenomena have been extensively studied in conventional materials, such as metals, ceramics and polymers [3] , [4] , [5] , [6] , [7] , the contribution of nanoscale morphologies to the high strain rate characteristics is still poorly understood. Polymers have recently attracted much attention because of their rate-dependent behaviours [8] and their ability to self-heal after projectile penetration [9] . In particular, polyurethane multiblock segmented copolymers, comprised of ‘hard’ and ‘soft’ domains assembled by preferential aggregation of polymer blocks consisting of glassy and rubbery segments display outstanding ballistic performance, and researchers have suggested that this could be a result of their nanoscale superstructures [10] , [11] . However, to date, the mechanical deformation of such superstructures at large strains and at high strain rates has not been directly studied at the nanoscale. Moreover, as exceptional mechanical performances have been recently discovered from artificially layered nanocomposites deformed at quasi-static rates [12] , [13] , [14] , [15] , extending high rate studies to the behaviour of layered nanocomposites is important, considering their significant potential as high-performance protective materials. In addition, at this scale, such nanocomposites may constitute a type of mechanical metamaterial, as the mechanical impedance periodicity is significantly smaller than the width of the impact-induced shock wave. Here, we provide the first detailed observations of model polymer layered nanocomposites subjected to hypervelocity projectile impacts. To visualize the entire deformation volume created by a high-speed impact, we introduce a microscopic ballistic test method using micron diameter glass spheres as bullets, which are fired to the sample by an energetic laser pulse and result in a deformation volume on the order of 1,000 μm 3 . Scanning electron microscopy (SEM) of focused ion beam cross-sections containing the projectile and the surrounding deformed material allow detailed study of a host of microstructural changes brought about by the impact event. Our investigation of nanomaterials via the microscopic ballistic test provides a new way to study high strain rate mechanical properties and can extend fundamental knowledge regarding the important role of nanostructures in protective materials. Depending on the orientation of the layers in the nanocomposite, the material responds to the impact with different deformation modes including layer kinking, layer compression, domain fragmentation and liquid formation by intermixing of the two polymer blocks. The compression-dominant response in the perpendicular impact to the layer orientation dissipates the impact energy more efficiently than the impact parallel to the orientation inducing the kinking-dominant response deformation with a 30% improvement in penetration depth, made possible by proper orientation of the layers. 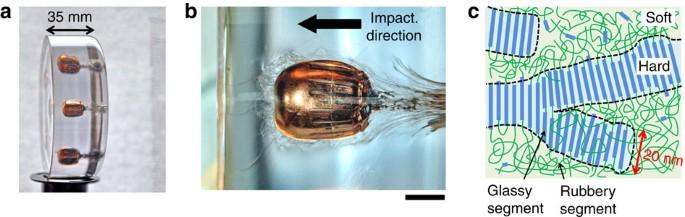Figure 1: Macroscopic ballistic impact test. (a) Photograph of a polyurethane disc (Cleargard, Courtesy of BAE Systems) impacted by copper jacketed 9 mm lead projectiles. (b) Magnified view of the projectile and penetration path. The scale bar is 5 mm. (c) Schematic of the nanostructure of a polyurethane nanocomposite comprised of glassy and rubbery domains. Macroscopic ballistic impact Figure 1a motivates our study—as shown in this image, a 35-mm thick polyurethane disc is able to arrest bullets travelling at ~350 m s −1 . The material shows complex deformation ahead of and around the embedded projectiles, including closing and healing of the projectile path without the presence of cracking or crazing that would render the material nontransparent (see Fig. 1b ). The detailed role of the hard glassy and soft rubbery domains (see Fig. 1c ) in absorbing the energy of the impact is unknown [10] , [11] . Figure 1: Macroscopic ballistic impact test. ( a ) Photograph of a polyurethane disc (Cleargard, Courtesy of BAE Systems) impacted by copper jacketed 9 mm lead projectiles. ( b ) Magnified view of the projectile and penetration path. The scale bar is 5 mm. ( c ) Schematic of the nanostructure of a polyurethane nanocomposite comprised of glassy and rubbery domains. Full size image Microscopic ballistic test and polymer nanocomposite To elucidate the types of deformation and failure events of polymer nanostructures that enable both the absorption of enormous impact energy as well as material recovery and healing, we utilize the laser-induced projectile impact test (LIPIT) illustrated in Fig. 2a . The details of LIPIT will be discussed in the Methods section. About 3.7 μm diameter silica beads (that is, μ-projectiles) impact and deform the nanostructured polymer specimen, and then cross-sectional imaging is used to directly visualize the μ-projectile and the surrounding deformation field. As a simple model layered composite system, we selected a polystyrene-polydimethylsiloxane (PS-b-PDMS) diblock-copolymer with block molecular weights of 22 and 24 kg mol −1 that approximates the usual microdomain sizes (5–20 nm) and mechanical impedance contrast in typical polyurethanes. Gel permeation chromatography shows that the block copolymer contains about 5% of homo-PS. The high temperature annealing treatment used to promote long range lamellar order and temperature rise during deformation likely cause some chain degradation which results in the presence of both homo-PS and homo-PDMS. Below its order–disorder transition temperature, the block copolymer self-assembles into a lamellar microphase-separated nanostructure. At ambient temperature and pressure and at low strain rates, PS is a ‘glassy’ polymer (glass transition temperature ( T g ) ~103 °C), elastic modulus (E~3.5 GPa) (ref. 16 ), whereas PDMS is a ‘rubbery’ polymer ( T g ~−125 °C, E~750 kPa) (ref. 17 ). Although both high strain rate [18] and high pressure [19] , [20] tend to increase the T g and modulus of polymers, the classification of glass and rubber is expected to remain valid at the impact of a μ-projectile because of the very low T g of PDMS and the large difference (230 °C) in T g of the respective blocks. This mechanical contrast is borne out via the observed microstructural deformation features (kink bands and the orientation dependence of the structure) that arise owing to the differences in the mechanical behaviour of the two types of blocks. Therefore, the glassy versus rubbery classification of the two polymers is still valid until the temperature rise due to the kinetic energy of an impact exceeds the elevated T g of the PS phase, when both blocks become fluid-like. As the elastic modulus of PS at ambient temperature and pressure is nearly 5,000 times larger than that of PDMS, the model PS-b-PDMS material is analogous to the ‘hard’ and ‘soft’ domains in the more complex mulitblock polyurethane materials depicted schematically in Fig. 1c . Macroscopic near-single-crystal glassy-rubbery layered block-copolymers are known to exhibit large mechanical anisotropy, hysteresis and good energy absorption under quasi-static testing [21] , [22] . Furthermore, the nanoscale domain structure of PS-b-PDMS is easily visualized by SEM owing to the higher secondary electron emission resulting from the silicon content of the (brighter) PDMS block (see Fig. 2b ). Further, because the layer periodicity, L 0 is two orders of magnitude smaller than the diameter of the μ-projectiles ( Fig. 2c ), the mechanical response of the material in our study will likely be characteristic of larger scale experiments. 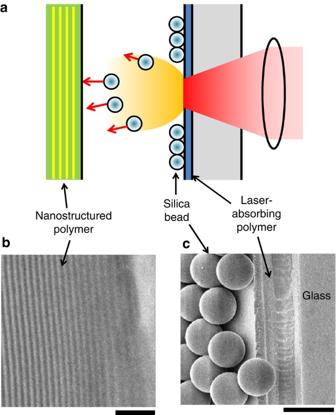Figure 2: Microscopic ballistic impact test (a) Scheme of the LIPIT. (b) Cross-sectional SEM image of a PS-b-PDMS lamellar target structure. The scale bar is 200 nm. (c) SEM images of the μ-projectiles on the absorbing polymer film before laser excitation. The scale bar is 5 μm. Figure 2: Microscopic ballistic impact test ( a ) Scheme of the LIPIT. ( b ) Cross-sectional SEM image of a PS-b-PDMS lamellar target structure. The scale bar is 200 nm. ( c ) SEM images of the μ-projectiles on the absorbing polymer film before laser excitation. The scale bar is 5 μm. Full size image Orientation-dependent deformation In this study, we investigate two microdomain orientations: parallel (H-) and perpendicular (V-) to the top surface of a sample. Approximating the penetration strain rate as v / h (ref. 23 ), where v and h are the initial impact velocity and depth of penetration, the estimated strain rate corresponding to a 1.1-km s −1 speed is on the order of 10 8 s −1 , higher than both conventional split-Hopkinson-pressure-bar (<10 5 s −1 ) (ref. 24 ) and ballistic nanoindentation (10 5 ~10 6 s −1 ) (ref. 25 ), which create large-area uniaxial compression and small linear local deformations, respectively. Furthermore, the LIPIT strain rate is comparable to deformation rates from explosively formed penetrators and micrometeorites (10 6 ~10 7 s −1 ) (ref. 26 ). After impact of the block copolymer by LIPIT, the temperature drops rapidly, freezing-in the deformation features as the PS block passes through its T g . To conduct post-impact analysis of this frozen state, high-resolution SEM images of focused ion beam milled cross-sections are taken on a plane containing the penetration axis and the mid-plane of the projectile, allowing for excellent microstructural characterization of the impacted volume (see Supplementary Fig. S1 ). As the initial nanostructures have well-defined L 0 and constant global orientation ( Fig. 2b ), the morphological changes in the cross-sectional images reveal the deformation and failure processes occurring during the high-speed impact and penetration. The overall deformation fields for three different projectile speeds (0.5, 1.1 and 1.5 km s −1 ) are visualized by colour-coded layer spacing-change maps, indicating layer dilation or compression ( Fig. 3a–c ) and colour-coded angular deviation maps ( Fig. 3d–f ), in which a large contrast in colour indicates a high degree of layer bending and kinking events. To create the high-resolution colour maps, angle and spacing values are calculated at each image pixel of the SEM images using Fourier transformation of a neighbourhood region (40 × 40 pixels) and a colour value corresponding the calculated spacing or angle is assigned to the pixel. 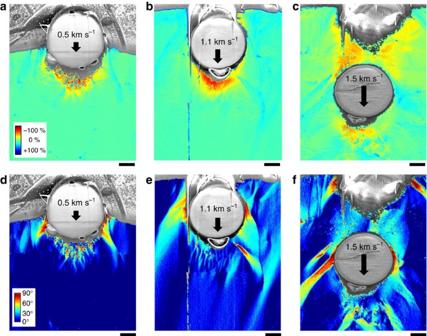Figure 3: Deformation of the H-lamellae targets for three velocities. (a–c) False colour maps of lamellar spacing on a logarithmic scale. (d–f) False colour maps of angular deviation from the original orientation on a linear scale. The colour mapping is not available for certain areas in which no periodicity exists or the resolution of image is insufficient. For fine features in the MZ, higher magnification SEM images are used for colour mapping around the MZ. Note the velocity dependent penetration depth and the presence of compressed layers (red-orange regions) behind the μ-projectile in (c). All scale bars are 1 μm. Figure 3: Deformation of the H-lamellae targets for three velocities. ( a – c ) False colour maps of lamellar spacing on a logarithmic scale. ( d – f ) False colour maps of angular deviation from the original orientation on a linear scale. The colour mapping is not available for certain areas in which no periodicity exists or the resolution of image is insufficient. For fine features in the MZ, higher magnification SEM images are used for colour mapping around the MZ. Note the velocity dependent penetration depth and the presence of compressed layers (red-orange regions) behind the μ-projectile in ( c ). All scale bars are 1 μm. Full size image The Mescall zone (MZ) [27] is the region directly ahead of a penetrator where the material experiences the most extreme conditions in temperature and pressure and the material behaviour here is primarily responsible for determining the penetration characteristics. Severely compressed lamellae are found in the MZ with up to 70% strain ( Fig. 3a ). The actual strain at the moment of impact is likely even higher because of some post-impact relaxation that occurs before quenching. Interestingly, for the largest projectile speed (1.5 km s −1 ) regions of highly compressed lamellae are found behind the μ-projectile, whereas less compressed lamellae are found in the MZ ( Fig. 3c ). In all impacts, kink bands are found at the sides of the penetration path. The lateral forces on the thin lamellar layers lead to the common kink-type shear band formation events seen in previous studies of slowly deformed (strain rates<1 s −1 ) single crystal bulk block-copolymers studied using in situ small-angle X-ray scattering [22] , [28] , [29] and/or postmortem transmission electron microscopy [30] . The slowest (0.5 km s −1 ) impact, shows kink bands near the surface created by an initial penetration of the μ-projectile ( Fig. 3d ), while Fig. 3e show additional kink bands in the MZ because of the lateral expansion of compressed lamellae from the volume displacement at the sides of the μ-projectile from deeper penetration of the higher velocity projectile. Local characteristics of energy absorbing deformation Detailed inspection of the SEM images of the MZ ( Fig. 4 ) shows that over the range of μ-projectile velocities studied, a strong evolution of the deformation features in the MZ occurs with projectile velocity. For 0.5 km s −1 , the layers in the MZ simply undergo severe compression ( Fig. 4a ) down to a period of about L 0 /3. The vertical compression in the MZ forces lateral expansion and leads to undulation of the lamellae at the periphery of the MZ. For the intermediate velocity of 1.1 km s −1 , we find in addition to the layer compression, domain fragmentation and just below the μ-projectile, the formation of an isotropic, sub-5 nm scale granular morphology ( Figs. 4b ). At the highest velocity (1.5 km s −1 ), with 10 times greater kinetic energy, there is an even finer scale, nearly homogeneous region adjacent to the μ-projectile in addition to the granular morphology region ( Fig. 4c ). Cavities are often found just below the μ-projectiles. As the rigid μ-projectile decelerates faster than the local polymer mass during elastic recoil it separates from the polymer mass at the front surface of the μ-projectile. Similar to the macroscopic polyurethane armour test in Fig. 1b , the μ-projectile penetration path is completely filled and sealed in the highest velocity, 1.5 km s −1 , impact ( Fig. 3c ). In the case of our model PS-b-PDMS material, the combination of elastic recovery of the laterally displaced material and flow of the fluid and fragmented layers heals the penetration path. Note the evidence of melted regions, relaxed but reoriented layers (with many disclination and dislocation type defects) and regions of highly compressed lamellae behind the projectile ( Fig. 5 ). 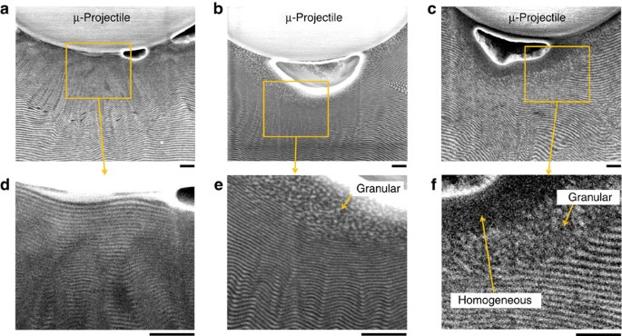Figure 4: Local deformation features. SEM images of the MZ for three different impact velocities, (a) 0.5 km s−1, (b) 1.1 km s−1and (c) 1.5 km s−1. (d–f) show × 3 magnified views of (a–c). All scale bars are 200 nm. Note the formation of granular isotropic and a homogeneous isotropic region at 1.1 and 1.5 km s−1. Figure 4: Local deformation features. SEM images of the MZ for three different impact velocities, ( a ) 0.5 km s −1 , ( b ) 1.1 km s −1 and ( c ) 1.5 km s −1 . ( d – f ) show × 3 magnified views of ( a – c ). All scale bars are 200 nm. Note the formation of granular isotropic and a homogeneous isotropic region at 1.1 and 1.5 km s −1 . 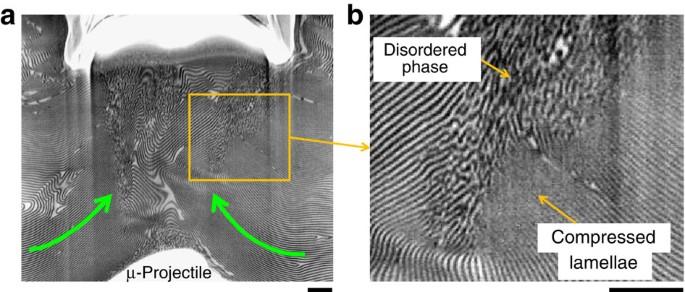Figure 5: Healing of the penetration path in the 1.5 km s−1impact. (a) Material flow (green arrows) and healing behind a μ-projectile. (b) A magnified view of the boxed region showing granular isotropic regions and highly compressed lamellae. Scale bars are 400 nm. Full size image Figure 5: Healing of the penetration path in the 1.5 km s −1 impact. ( a ) Material flow (green arrows) and healing behind a μ-projectile. ( b ) A magnified view of the boxed region showing granular isotropic regions and highly compressed lamellae. Scale bars are 400 nm. Full size image The influence of the orientation of the nanostructure on penetration and deformation was assessed by impact at an intermediate speed (1.1 km s −1 ) using lamellae in the V-orientation. The spacing and angular deviation maps ( Fig. 6a ) reveal that the lamellae in the MZ undergo strong reorientation events via kinking without the lamellar compression observed for the H-lamellae ( Fig. 3b ). These kink bands extend a significant distance below the μ-projectile, considerably further than the deformation zone for the H-lamellae. The SEM images of the MZ ( Fig. 6c ) show that the lamellae in the MZ undergo shear localization and extensive kinking leading to chevron and omega lamellar tilt boundaries. Moreover, as similar kinking features are observed when deforming mechanically heterogeneous layers in quasi-static deformation [31] , we can infer that there is sufficient mechanical contrast during this high strain rate deformation event despite rate-dependent molecular motions and temperature rise because of the adiabatic compression. As the μ-projectile penetrates, the kink bands become thinner owing to greater layer reorientation. In the more severely deformed regions, layer undulation and compression lead to domain fragmentation. Closest to the μ-projectile, a small region of the isotropic granular structure is formed, but is less extensive in size compared with similar regions in the H-lamellae targets. 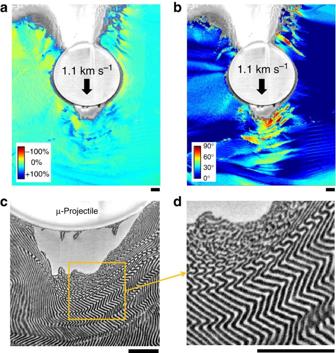Figure 6: High strain rate responses of the V-lamellae against penetration of a 1.1-km s−1μ-projectile. (a) False colour map of lamellar spacing on a logarithmic scale. (b) False colour map of angular deviation from the original orientation on a linear scale (c) SEM image of the MZ shows multiple kink bands below the μ-projectile and a cavity that filled with homo-PDMS. (d) Magnified view of the boxed area in (c) showing the granular phase and omega boundaries. All scale bars are 500 nm. Figure 6: High strain rate responses of the V-lamellae against penetration of a 1.1-km s −1 μ-projectile. ( a ) False colour map of lamellar spacing on a logarithmic scale. ( b ) False colour map of angular deviation from the original orientation on a linear scale ( c ) SEM image of the MZ shows multiple kink bands below the μ-projectile and a cavity that filled with homo-PDMS. ( d ) Magnified view of the boxed area in ( c ) showing the granular phase and omega boundaries. All scale bars are 500 nm. Full size image First we focus on the surprising observation that the significant layer deformation in the MZ can lead to ‘melting’ and intermixing of the two types of block layers. The small granular features ( Fig. 4e ) are domain fragments and local compositional fluctuations, whereas the more homogeneous region ( Fig. 4f ) corresponds to a quenched-in homogeneous disordered melt [32] , [33] induced by the mechanical energy input of the nearly adiabatic compression. The existence of these disordered regions is remarkable as the order–disorder transition temperature at ambient pressure of this strongly segregated PS-b-PDMS system is estimated to be over 3,000 °C—much greater than the material decomposition temperature (265~280 °C) (ref. 34 ). An estimate of a temperature rise is problematic because of the strong gradients in the deformation and the uncertainty in the material’s heat capacity( T , P ) and the efficiency of energy conversion but the rise could be 100 to 1,000 s of degrees Celsius depending on the assumptions, so it may be possible for the kinetic energy deposition to raise the temperature above the order–disorder transition temperature. We approximate the pressure of lamellae near the MZ at the initial impact moment by the Rankine–Hugoniot relation [35] derived from the conservation of momentum, where ρ 0 , U s , and u p are an initial density, shock velocity and particle velocity (or local mass velocity) of the block copolymer. As Carter and Marsh observed [4] , there is a linear relation between shock velocity and particle velocity for polymers, where c 0 and s are the average sound velocity in the material and an empirical linear fitting parameter. Thus, we can estimate the pressure for a range of the impact speeds using ρ 0 =0.97 g cm −3 (ref. 36 ), c 0 =1.03 km s −1 (ref. 37 ), and s =1.54 (ref. 38 ) for PDMS, ρ 0 =1.03 g cm −3 , c 0 =2.21 km s −1 , and s =1.84 for PS (ref. 39 ), and ρ 0 =2.15 g cm −3 , c 0 =2.97 km s −1 and s =0.84 for quartz [40] . From equations (1) and (2), the estimated pressures in the MZ are 0.8, 2.3 and 3.2 GPa for impact speeds of 0.5, 1.1 and 1.5 km s −1 , respectively. As illustrated in Fig. 7a , therefore, the initial structure is severely compressed and this mechanical compression significantly increases the free energy of the lamellar structure owing to both the increased number of enthalpically unfavourable layer interfaces per unit volume and the entropically unfavourable penalty for severely pancaked chain conformations within the layers. To reduce the energy, the ordered domains fragment, the chains relax and mix into a granular disordered phase at an elevated temperature (at least higher than the effective T g of PS—see Fig. 7 ). As the temperature goes even higher, the granular phase evolves to the homogeneous phase by further segmental mixing. Post-impact annealing experiments show that the block copolymer has not substantially degraded/crosslinked during the brief temperature excursion as all of the homogeneous and fragmented regions revert to long range ordered lamellae with the original 40 nm period (see Supplementary Fig. S2 ). The transformation of the layered structure into a combination of liquid and highly compressed layers absorbs a larger amount of the impact energy per unit volume of material than the dominant kinking mechanism observed for the V-lamellae. 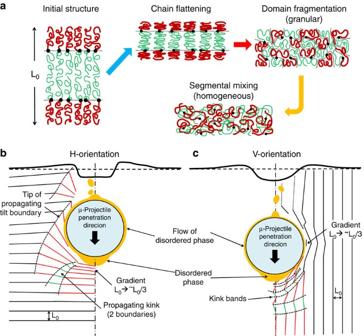Figure 7: Schematic of various deformation features. (a) Illustration of mechanically driven transformation into a fragmented and segmentally mixed fluid phase. Characteristics of deformation of (b) H-lamellae and (c) V-lamellae. The orange colour shows regions around the projectile that transformed into granular or homogeneous fluid. Figure 7: Schematic of various deformation features. ( a ) Illustration of mechanically driven transformation into a fragmented and segmentally mixed fluid phase. Characteristics of deformation of ( b ) H-lamellae and ( c ) V-lamellae. The orange colour shows regions around the projectile that transformed into granular or homogeneous fluid. Full size image In Fig. 7b , simplified deformation scenarios for the H- and V- lamellae are depicted based on evidence from the deformation colour maps of H-lamellae in Fig. 3 and those of V-lamellae in Fig. 6 . For the H-lamellae ( Fig. 7b ), as the μ-projectile contacts the material, the lamellae in the MZ directly ahead of the μ-projectile become severely uniaxially compressed and mechanical energy absorption elevates the temperature over the T g of the PS layers. Together with the temperature rise, the compressed layer structure fragments and both a fragmented and a homogenous phase form if the magnitude of the adiabatic compression is sufficient (order of GPa). The liquid regions act as a lubricant and provide for block-copolymer material to flow around the advancing μ-projectile. In addition, the extreme shear forces [41] experienced as the polymer melt flows around the surface of penetrating μ-projectile may promote the additional disordering/mixing of the microphase-separated melt. As the μ-projectile penetrates deeper, the fluid reaches the distal portion of the μ-projectile and together with the elastically compressed lateral material rapidly relaxes to fill in and heal the gap behind the μ-projectile. In contrast, the response of V-lamellae ( Fig. 7c ) begins with kink band formation mostly on the line of penetration. This behaviour creates a more extensive deformation volume than that of the H-lamellae. As the deviation of angle becomes larger at the proximate region of the μ-projectile, lamellae compression and fine scale fragmentation of the lamellae create some fluid. From the μ-projectile penetration depth versus velocity data, we observe that the H-lamellae stop the projectiles significantly better than the V-lamellae. For example, at a velocity of 1.1 km s −1 , the H-lamellae stop the μ-projectile in a distance of 4.2±0.7 μm (from ten events) versus 6.1±0.9 μm for the V-lamellae (from twelve events). Note that the deepest position of the μ-projectile at each impact is likely to be more than the measured depth owing to elastic recoiling of the material and projectile, so that it is possible that the material immediately below the projectile position is itself wake material. This is consistent with the observation of a larger volume of the disordered phase for the H-lamellae, as the shorter stopping distance means higher pressure and temperature (more favourable conditions to create the disordered fluid phase). Consequently, the different penetration depths imply that the compression-dominant high strain rate responses of the H-lamellae are more efficient at resisting the penetration than the disorientation-dominant high strain rate response of the V-lamellae. In practical terms, choice of the H-orientation would advantageously decrease the armour thickness (areal density) by 30%, for protection against a given threat. Interestingly, the static modulus of the V-lamellae is about 3 times higher than that of the H-lamellae and absorbs more energy in quasi-static deformation [22] ; thus, this opposite behaviour in the high strain rate deformation should arise from the dynamic compression processes of the H-lamellae. For uniaxial compression, the ratio between the mechanical impedances ( ) of PS and PDMS is quite large (~70). In the macroscopically periodic layered composite consisting of alternating hard and soft layers, propagating shock waves have been demonstrated to undergo multiple reflections because of the mechanical impedance mismatch, and these reflections reduce the propagation velocity of the shock waves, and thereby enhance dissipation of the shock energy [42] . Considering the very thin nature of the H-lamellae, reflected shock waves can nearly immediately affect the penetrating μ-projectile within 30 ps (~ L 0 / c 0 ) and transfer their momentum in the opposite direction of the penetration. In contrast for the V-lamellae, almost no shock wave coupling occurs because of the wave propagation is parallel to the lamellar interfaces. As the overall microdomain morphology of a polyurethane is usually isotropic, both shock wave coupling and segmental mixing effects can similarly enhance the protection material performance. Two counterintuitive observations are the smaller layer compression in the MZ ( Fig. 4f ) and the highly compressed region behind of the μ-projectile ( Figs 3c and 5b ). One possible scenario is that the high pressure and compression in front of the penetrator cause the layer compression and as the material is pushed to the side, the temperature and stress level drops and the layers become frozen in their compressed state. The projectile moves forward, pushes the compressed material to the side and eventually these compressed regions relax back behind the advancing projectile with some regions having cooled sufficiently rapidly to maintain some layer compression. In this scenario, the plasticity largely occurs in the MZ, then is retained as the material is displaced sideways and remains frozen in the infilled region behind the μ-projectile with the fluid ‘gluing’ the lamellar regions together. In summary, the mechanical responses of model glassy-rubbery nanostructured layered polymer materials at large strain and high strain rate are revealed at high spatial resolution. The lamellar nanocomposite absorbs the kinetic energy of a hypervelocity incident μ-projectile via layer kinking, layer compression, extreme chain conformational flattening, domain fragmentation and ultimately segmental mixing, leading to mechanical ‘melting’ of the initially well-ordered material. The shock wave coupling effect arising from nanoscale mechanical layer impedance contrast can also enhance energy dissipation. Although detailed correspondence of our micro-ballistic test to macroscopic tests will be assessed in the future, our approach using LIPIT allows facile study of the high strain rate mechanical responses of other interesting light weight nanostructured materials, such as boron nitride, carbon nanotube reinforced composites, graphite and graphene layers and their nanocomposites with polymer matrices and metal substrates, and should extend fundamental understanding and bring about new nanostructured materials for improved ballistic performance under extreme mechanical conditions. Preparation of μ -projectiles A laser absorbing dye (Epolight 3036, Epolin Inc.), polystyrene (MW 800~5,000 g mol −1 , Polyscience Inc.) and propylene glycol methyl ether acetate (Sigma Aldrich) used as received are mixed with a weight ratio of 1:10:30 and spin-coated onto a glass substrate (corning no. two microscope cover slip) at 1,000 r.p.m. for 2 min to form a 3.8-μm thick layer. This layer absorbs ~98% of the light at 800 nm. Next 3.7 μm diameter solid silica beads (Microparticles GmbH) are exposed to hexamethyldisilazane vapour under a low vacuum for 30 min to render their surface hydrophobic. A 5 wt% ethanol suspension of the treated beads is then dropped on a water surface to float a monolayer of the beads, and the monolayer is transferred to the polymer-coated glass substrate by making contact with the glass substrate. 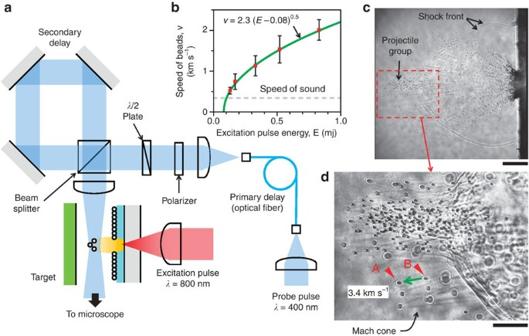Figure 8: Laser-induced projectile impact test. (a) Diagram of the optical setup for LIPIT. (b) The speed of the μ-projectiles is proportional to the square root of the excitation pulse energy for a given thickness of the absorbing polymer layer. The error bar represents the maximum and minimum speeds for each median value and the green line is a fitting curve. (c) Double exposure photograph with a 22-ns interval at 250 ns after the excitation laser pulse. The scale bar is 200 μm. (d) Expanded section of (c). Here, each μ-projectile appears twice; for example, the μ-projectile marked as ‘A’ is the same μ-projectile marked as ‘B’ and the corresponding speed is 3.4 km s−1. Only the μ-projectiles outside of the shock front present a Mach cone, appearing when an object’s speed exceeds the speed of sound. The sizes of the μ-projectiles appear differently depending on their distance to the microscope objective lens. The scale bar is 100 μm. Laser-induced projectile impact test Figure 8a shows the optical configuration for LIPIT. An excitation laser pulse (300 ps pulse duration, 800 nm wavelength) is created by a pulsed laser system consisting of an optical parametric oscillator (MTS Mini Ti:sapphire Laser Kit, Kapteyn–Murnane Laboratories L.L.C) pumped by a diode pumped solid state laser (Verdi V6, Coherent) with a Ti:sapphire amplifier (Titan, Quantronix Inc.). A monolayer of the μ-projectiles on a laser absorbing polymer-coated glass substrate ( Fig. 2c ) can be accelerated to speeds of up to 4 km s −1 by rapid expansion of gas produced by the laser ablation when a single pulse is focused by a 30-mm focal length lens. The synchronized probe pulse (250 fs pulse duration, 400 nm wavelength) is delayed ~250 ns by use of a 50-m long multimode optical fibre and split into two pulses. One of the two pulses is additionally delayed for 22 ns by the secondary optical path in air and both pulses are collimated by a 50-mm focal length condenser lens to image the flying μ-projectiles. Figure 8c shows images of 3.7 μm diameter μ-projectiles moving toward a sample. The excitation laser pulse generates a supersonic gas plume surrounded by a shock front trailed by the μ-projectiles. Deceleration of the μ-projectiles by air is negligible until the μ-projectiles overtake the shock front, as evidenced by the appearance of individual Mach cones ( Fig. 8d ). Therefore, by placing a target sample at a position where the shock front arrives before the μ-projectiles (here 700 μm), the flight speed can be used as the impact speed. As demonstrated in Fig. 8b , the kinetic energy of the μ-projectiles is linearly proportional to the input energy after subtracting the energy used for polymer ablation (0.08 mJ). LIPIT allows a compact test specimen size enabling high resolution investigation of the entire deformation/failure zone in prototype nanostructured materials (which often are only initially available as small samples), control of the kinetic energy (for example, projectile velocity), and enables a wide choice of projectiles regardless of their conductivity, shape and size, compared with electrostatic accelerator [43] , Van der Graaff linear accelerator [44] and laser driven flyer techniques [45] by virtue of its indirect acceleration mechanism. Moreover, the indirect means is advantageous to avoid any laser irradiation damage when using delicate projectiles made of polymers and bio-substance as observed in the laser-induced forward transfer technique [46] . We have recently completed the development of an advanced LIPIT apparatus, which can fire a single μ-projectile and take a triple exposure photograph, such that the error in velocity can be reduced below 4% and the instantaneous acceleration information can be acquired. Figure 8: Laser-induced projectile impact test. ( a ) Diagram of the optical setup for LIPIT. ( b ) The speed of the μ-projectiles is proportional to the square root of the excitation pulse energy for a given thickness of the absorbing polymer layer. The error bar represents the maximum and minimum speeds for each median value and the green line is a fitting curve. ( c ) Double exposure photograph with a 22-ns interval at 250 ns after the excitation laser pulse. The scale bar is 200 μm. ( d ) Expanded section of ( c ). Here, each μ-projectile appears twice; for example, the μ-projectile marked as ‘A’ is the same μ-projectile marked as ‘B’ and the corresponding speed is 3.4 km s −1 . Only the μ-projectiles outside of the shock front present a Mach cone, appearing when an object’s speed exceeds the speed of sound. The sizes of the μ-projectiles appear differently depending on their distance to the microscope objective lens. The scale bar is 100 μm. Full size image Preparation of self-assembled polymer samples To make a 0.5~1 mm thick self-assembled polymer film, a 10 wt% toluene solution of PS-b-PDMS is drop-cast onto a previously crosslinked PDMS (Sylgard 184, Dow Corning) substrate. The PDMS substrate creates PDMS preferential wetting and an H-oriented lamellar structure. Thermal annealing at 150 °C for 24 h under vacuum eliminates some defects and promotes long range order. The annealed PS-b-PDMS film having the layers parallel to the substrate is then mechanically delaminated from the PDMS substrate and the bottom surface is used as the impact surface for the H-orientation experiment. For the V-orientation experiment, the annealed sample is fractured perpendicular to the lamellae in liquid nitrogen and the fractured surface is used for the impact surface as its roughness is small enough compared with the size of the μ-projectile. How to cite this article: Lee J.-H. et al . High strain rate deformation of layered nanocomposites. Nat. Commun. 3:1164 doi: 10.1038/ncomms2166 (2012).